Charge stripe order near the surface of 12-percent doped La2−xSrxCuO4 A collective order of spin and charge degrees of freedom into stripes has been predicted to be a possible ground state of hole-doped CuO 2 planes, which are the building blocks of high-temperature superconductors. In fact, stripe-like spin and charge order has been observed in various layered cuprate systems. For the prototypical high-temperature superconductor La 2− x Sr x CuO 4 , no charge-stripe signal has been found so far, but several indications for a proximity to their formation. Here we report the observation of a pronounced charge-stripe signal in the near surface region of 12-percent doped La 2− x Sr x CuO 4 . We conclude that this compound is sufficiently close to charge stripe formation that small perturbations or reduced dimensionality near the surface can stabilize this order. Our finding of different phases in the bulk and near the surface of La 2− x Sr x CuO 4 should be relevant for the interpretation of data from surface-sensitive probes, which are widely used for La 2− x Sr x CuO 4 and similar systems. High-temperature superconductivity occurs in copper oxide systems that crystallize in a layered perovskite structure. The characteristic building blocks of these systems are well-separated copper-oxide planes ( Fig. 1a ). In the parent compound of the single-layered cuprate superconductors, La 2 CuO 4 , the Cu 2+ ions in these planes carry a spin ( S =1/2) and couple antiferromagnetically. Chemical doping by replacing trivalent La with alkaline earth like Ba or Sr introduces holes into the system. Doping holes in the CuO 2 planes has been suggested to lead to the formation of non-magnetic Zhang-Rice singlets [1] suppressing the local moment at the individual Cu sites. As the free mobility of holes in a two-dimensional antiferromagnetic matrix is energetically not favourable, the formation of stripes was postulated [2] , [3] , [4] , [5] , in which hole-rich, non-magnetic sites form one-dimensional lines acting as anti-phase domain walls for the antiferromagnetic order on the hole-poor sites ( Fig. 1b ). Such an arrangement allows holes to hop along the stripes as well as transversal hopping of the whole stripe and avoids magnetic frustration. In the pseudo-gap phases of HgBa 2 CuO 4+δ (Hg1202) [6] , [7] , YBa 2 Cu 3 O 6 [8] and under-doped La 2− x Sr x CuO 4 (LSCO) [9] , signatures of another order parameter have been reported with properties as predicted in the orbital-current model [10] . It was proposed that this other order competes with stripe order and that its suppression results in a suppression of high-temperature superconductivity [9] . 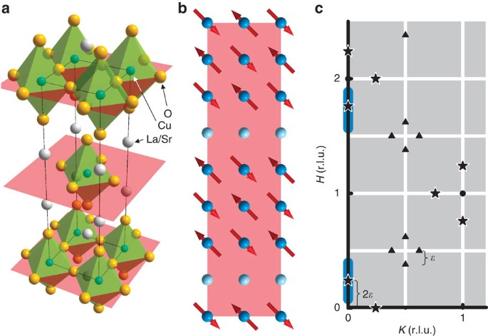Figure 1: Stripe order and the observed charge-order peaks. (a) Crystal structure of the layered perovskite cuprates and nickelates. (b) A model picture of site-centred stripe order in the CuO planes (red planes in panel (a)) where only the Cu sites are shown. Light blue denotes hole-rich, dark blue hole-poor sites; the arrows indicate the spin direction. (c) Reciprocal space map with fundamental Bragg peaks (filled circles) and spin order (triangles) and charge-order (stars) superstructure reflections related to the stripe phase. The blue lines denote the direction of the scans presented inFig. 2. Figure 1: Stripe order and the observed charge-order peaks. ( a ) Crystal structure of the layered perovskite cuprates and nickelates. ( b ) A model picture of site-centred stripe order in the CuO planes (red planes in panel ( a )) where only the Cu sites are shown. Light blue denotes hole-rich, dark blue hole-poor sites; the arrows indicate the spin direction. ( c ) Reciprocal space map with fundamental Bragg peaks (filled circles) and spin order (triangles) and charge-order (stars) superstructure reflections related to the stripe phase. The blue lines denote the direction of the scans presented in Fig. 2 . Full size image Experimentally, stripes were first observed in layered nickelates [11] , [12] . Stripes in cuprate systems were observed in the low-temperature tetragonal (LTT) phases of La 2− x − y Nd y Sr x CuO 4 (LNSCO) [13] , [14] , [15] , [16] , La 2− x Ba x CuO 4 (LBCO) [17] , La 2− x − y Eu y Sr x CuO 4 (LESCO) [18] in neutron and in X-ray diffraction experiments [19] . Recently, stripe order was found in layered cobaltates [20] . In reciprocal space, the charge order (CO) and the spin order (SO) in a stripe phase lead to different, well-separated superstructure reflections: CO reflections occur in a distance 2 around fundamental Bragg peaks, whereas SO reflections are split off by half of that distance, that is, , from the (½,½) antiferromagnetic positions of the undoped phase ( Fig. 1c ). The value of depends on the amount of doping [21] . In contrast to a coupled spin-density wave and charge-density wave as found, for example, in chromium metal [22] , the stripe phase is further characterized by a higher transition temperature for CO than for SO owing to the two-dimensional character of the magnetic order [23] . For the prototypical high-temperature superconductor LSCO, no charge-stripe signal has been found so far [19] , [24] . On the other hand, several indications for the proximity to a stripe phase exist: a weak static stripe-like SO signal for doping levels below 0.15 has been observed [25] , [26] as well as magnetic correlations indicating fluctuating magnetic stripes with the characteristic relation between doping level and stripe spacing [21] . Although no spatial modulations of the Cu–O bond lengths, which are indicative for charge order, were observed for LSCO, the softening and broadening of the corresponding bond-stretching phonon mode was interpreted as a precursor for the formation of charge stripes [27] . The occurrence of static charge-stripe ordering in LNSCO, LBCO and LESCO has been attributed to the LTT symmetry of the respective phases, where tilting around the Cu–O bonds generates two distinct in-plane oxygen sites. The LTT tilt pattern is thus likely to stabilize stripe order; it is less clear, however, if it is required. In fact, for La 1.875 Ba 0.125− x Sr x CuO 4 stripe-like charge order has been observed in the low-temperature orthorhombic (LTO) phase in vicinity to the low-temperature less orthorhombic (LTLO) phase most likely due to enhanced structural disorder [28] . We show in the following that charge stripes develop in the near-surface region of 12-per cent doped LSCO, but not in the bulk. Approach We studied pieces from the same single crystal of 12-per cent doped LSCO with 2 techniques: resonant soft X-ray diffraction (RSXD), which is moderately surface sensitive with a probing depth of several nanometres, and high-energy X-ray diffraction, which is bulk sensitive with a probing depth of several millimetres. Both techniques are sensitive to charge stripes: RSXD uses the high spectroscopic sensitivity of dipole-allowed excitations into oxygen 2 p and transition-metal 3 d states to the electronic state of the scattering ions to probe spatial modulations of these states in a diffraction experiment [17] , [18] , [29] , [30] . High-energy X-ray diffraction probes the lattice distortion related to charge order [16] and allows to detect superstructure reflections that are more than eight orders of magnitude weaker than fundamental Bragg peaks. Charge stripes near the surface In the RSXD experiment, we find a clear peak at the CO position (h 0 0), h ≈0.24, at the oxygen 1 s →2 p ( K , black curve in Fig. 2a ) as well as at the copper 2 p →3 d ( L 2,3 ) resonances. To identify the electronic character of the peak, we compare its energy dependence with that from an equally doped sample of La 1.48 Nd 0.4 Sr 0.12 CuO 4 (LNSCO, red curve in Fig. 2a ) for which the existence of static charge stripes has been established by neutron and X-ray diffraction [13] , [14] , [15] , [16] . The resonance spectra, that is, the energy dependences of the peak intensity across the resonances are displayed in Fig. 3, together with X-ray absorption spectroscopy data. The resonance spectra are very similar for both systems and resemble those published for charge-order peaks in LBCO [17] and in LESCO [18] , thus proving that charge-stripe order is the common electronic origin of all peaks. The assignment of the LSCO (0.24 0 0) peak to charge-stripe order is further confirmed by its temperature dependence. The decay of the LSCO (0.24 0 0)-peak intensity on heating is displayed in Fig. 4a . The peak vanishes around 55 K. For comparison, the susceptibility is plotted ( Fig. 4b ), which shows a critical temperature for superconductivity at T c =30 K. From neutron scattering experiments using a sample with very similar composition, it is known that the very weak magnetic ordering melts at about the same temperature as superconductivity [25] , which is much lower than what we find for the disappearance of the (0.24 0 0) peak.This behaviour with T CO > T N is exactly what is expected for stripe order in layered cuprates [23] . 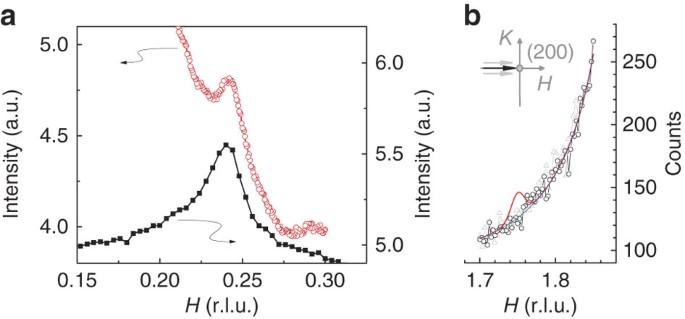Figure 2: Reciprocal space scans through charge-order positions. (a) Scans along [100] (H) through the (0.24 0 0) superstructure peaks for LSCO (black filled symbols) and LNSCO (red open symbols) recorded at the O–Kresonance with the samples held at 18 K. The shape of the background is different, but the peaks are clearly visible and of similar intensity. The correlation length alongafor LSCO, as determined from the peak width, is about 40 Å (≈10 Cu–Cu distances) comparable to that observed for LNSCO (≈50 Å). (b) Example for high-energy X-ray scans through an expected charge-order satellite position near (200) (symbols and blue line) and slightly offset inK(grey symbols) to be sure not to miss any signal. The red line is a simulation of a charge-order peak at what we estimate to be our detection limit, which is of the order of 10−8times the intensity of a strong nuclear reflection; note that the width of this simulation corresponds to that seen in the RSXD experiment. Figure 2: Reciprocal space scans through charge-order positions. ( a ) Scans along [100] ( H ) through the (0.24 0 0) superstructure peaks for LSCO (black filled symbols) and LNSCO (red open symbols) recorded at the O– K resonance with the samples held at 18 K. The shape of the background is different, but the peaks are clearly visible and of similar intensity. The correlation length along a for LSCO, as determined from the peak width, is about 40 Å (≈10 Cu–Cu distances) comparable to that observed for LNSCO (≈50 Å). ( b ) Example for high-energy X-ray scans through an expected charge-order satellite position near (200) (symbols and blue line) and slightly offset in K (grey symbols) to be sure not to miss any signal. The red line is a simulation of a charge-order peak at what we estimate to be our detection limit, which is of the order of 10 −8 times the intensity of a strong nuclear reflection; note that the width of this simulation corresponds to that seen in the RSXD experiment. 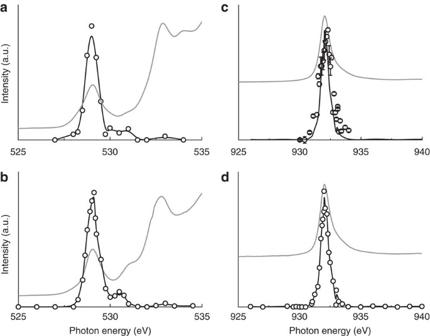Figure 3: Resonance spectra from LSCO and LNSCO. Energy dependence of the (0.24 0 0) RSXD signals (symbols) as observed at the oxygen 1s→2p(O–K) resonance for LSCO (a) and LNSCO (b) and at the copper 2p3/2→3d(L3) resonance for LSCO (c) and LNSCO (d). The black lines through the symbols are guides to the eye; for comparison, these lines are identical in (c) and (d). The respective X-ray absorption signals (grey line) are shown as energy references. Full size image Figure 3: Resonance spectra from LSCO and LNSCO. Energy dependence of the (0.24 0 0) RSXD signals (symbols) as observed at the oxygen 1 s →2 p (O– K ) resonance for LSCO ( a ) and LNSCO ( b ) and at the copper 2 p 3/2 →3 d ( L 3 ) resonance for LSCO ( c ) and LNSCO ( d ). The black lines through the symbols are guides to the eye; for comparison, these lines are identical in ( c ) and ( d ). The respective X-ray absorption signals (grey line) are shown as energy references. 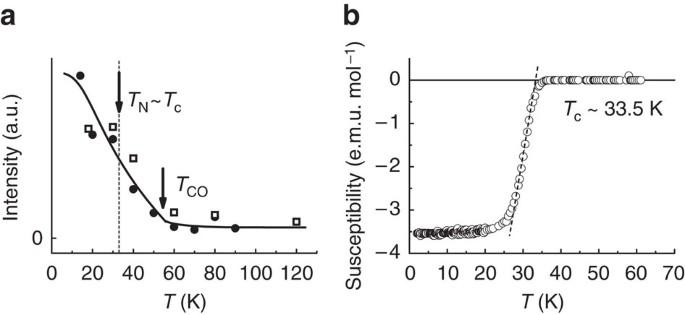Figure 4: Temperature dependence. (a) Temperature dependence of the (0.24 0 0) RSXD signal in LSCO as recorded at the Cu-L3(filled symbols) and O–Kresonance (open symbols). (b) Susceptibility, which indicates superconductivity below 30 K. The (0.24 0 0) signal is observable up to about 55 K ruling out a magnetic origin of this peak. Full size image Figure 4: Temperature dependence. ( a ) Temperature dependence of the (0.24 0 0) RSXD signal in LSCO as recorded at the Cu- L 3 (filled symbols) and O– K resonance (open symbols). ( b ) Susceptibility, which indicates superconductivity below 30 K. The (0.24 0 0) signal is observable up to about 55 K ruling out a magnetic origin of this peak. Full size image No charge stripes in the bulk Our RSXD experiment shows clearly the existence of charge-stripe order in 12-per cent doped LSCO. On the other hand, in our high-energy X-ray diffraction data, no trace of charge order can be found. We scanned at various possible charge-order positions without any positive results. An example scan is presented in Fig. 2b . Combining these two results, we conclude that charge-stripe order does exist in the near-surface region of LSCO but not in the bulk. From the RSXD peak profile, we determine the coherence length of charge order perpendicular to the (100)-oriented surface to be at least in the range between 4 and 6 nm. This is shorter than the probing depth at the oxygen- K resonance and hence gives a lower limit for the thickness of the charge-ordered surface region. The sensitivity of the high-energy X-ray diffraction experiment was high enough to exclude a possible scenario of such short-range-correlated charge order in the whole sample volume. We only find it near the surface. Surface-preparation effects To clarify whether strain caused by polishing induced charge order, we carried our RSXD experiments from in-situ cleaved samples. For these a (001) surface orientation is determined by the cleavage plane of LSCO and (0.24 0 0) is not accessible. From other cuprates, it is known that the charge-order peak is visible over a wide range of L-values [16] and indeed, we found a charge-order signal at (0.24 0 ℓ) with 0.65≤ℓ≤0.8, which exhibits the same dependence on temperature and energy as the (0.24 0 0) peak from the (100)-oriented samples. The occurrence of charge order in LSCO is hence neither a property of a particular surface nor is it induced by a particular surface preparation method. It is an intrinsic property of the near-surface region, where reduced dimensionality or structural relaxations apparently stabilize an order, which does not form in the bulk. We note that we did not find any signal from charge stripes in a surface-sensitive RSXD experiment from a 14-per cent doped LSCO sample. The observation of stabilized charge order in the near-surface region of 12-per cent doped LSCO is surprising, as one usually expects a three-dimensional crystal to start melting at the surface. We tentatively attribute the enhanced stability of the charge ordering at the surface to the documented impact of disorder on local tilting and on electronic mobility. The structural disorder should be larger at the surface and it induces charge ordering in the La 1.875 Ba 0.125− x Sr x CuO 4 series. In nickelates [31] and in manganates [32] , also, disorder stabilizes stripe or other types of charge-ordered phases. The fact that the near-surface region of LSCO is different from the bulk should be considered when surface-sensitive experiments from LSCO and related systems are interpreted in terms of bulk properties of the material. Stripes are known to affect the shape of the Fermi surface as seen in angle-resolved photoemission experiments [33] , [34] , [35] , [36] . Our finding may, for example, help to relate the apparent similarities in the Fermi-surfaces of LNSCO [34] and LSCO [35] to the different superconducting properties of these compounds. In scanning tunnelling spectroscopy experiments, spatial modulations of the local density of states have been observed for different cuprate systems [37] , [38] . For 12-per cent doped LSCO spatial modulations on different length scales have been observed [39] ; for the interpretation of these, the existence of charge stripes may matter [40] . In conclusion, RSXD experiments prove the existence of charge-stripe order in an at least 4-nm thick, near-surface region of 12-per cent doped LSCO, while at the same time, there is no indication for such kind of order in the bulk. The near-surface order does not depend on the surface orientation and preparation method, but seems to be an intrinsic property of the surface. The well-established proximity of LSCO to the formation of charge stripes is apparently sufficient to drive the phase transition near the surface. Samples Single crystals of La 1. 88 Sr 0.12 CuO 4 and La 1.48 Nd 0.4 Sr 0.12 CuO 4 were prepared by floating-zone method using an image furnace. The indexation of reciprocal space points refers to the high-temperature tetragonal unit cell with a ≈3.78 Å and c ≈13.2 Å. Resonant soft X-ray diffraction and X-ray absorption The RSXD measurements were carried out at UE46-PGM-1 beamline at the synchrotron-radiation source BESSY II operated by the Helmholtz-Zentrum Berlin. The two-circle ultrahigh vacuum diffractometer designed at Freie Universität Berlin was used in horizontal scattering geometry. The polarization vector of the incoming X-rays was perpendicular to the scattering plane, and parallel to the b axis of the single crystals. For the RSXD experiment, two different sample orientations were used: samples with a (100) surface normal were polished ex situ ; those with a (001) surface normal were cleaved in situ . The energy dependence of the diffraction features was determined by taking scans along [100] through the peak (similar to Fig. 2a ) for every photon energy. The X-ray absorption spectroscopy spectra were obtained from the total-electron yield signal recorded as the sample drain current. The energy resolution of X-rays near the oxygen K edge and the copper L edge are ~90 and 210 meV, respectively. High-energy X-ray diffraction and susceptibility High-energy X-ray diffraction experiments were carried out at beamline BW5 at DESY using 100 keV X-rays. Susceptibility measurements were carried out in a field of 50 Oe after zero-field cooling using a small piece of the same single crystal as used for the diffraction experiments. How to cite this article: Wu, H.-H. et al . Charge stripe order near the surface of 12-per cent doped La 2− x Sr x CuO 4 . Nat. Commun. 3:1023 doi: 10.1038/ncomms2019 (2012).